Plant immune response to pathogens differs with changing temperatures Temperature fluctuation is a key determinant for microbial invasion and host evasion. In contrast to mammals that maintain constant body temperature, plant temperature oscillates on a daily basis. It remains elusive how plants operate inducible defenses in response to temperature fluctuation. Here we report that ambient temperature changes lead to pronounced shifts of the following two distinct plant immune responses: pattern-triggered immunity (PTI) and effector-triggered immunity (ETI). Plants preferentially activate ETI signaling at relatively low temperatures (10–23 °C), whereas they switch to PTI signaling at moderately elevated temperatures (23–32 °C). The Arabidopsis arp6 and hta9hta11 mutants, phenocopying plants grown at elevated temperatures, exhibit enhanced PTI and yet reduced ETI responses. As the secretion of bacterial effectors favours low temperatures, whereas bacteria multiply vigorously at elevated temperatures accompanied with increased microbe-associated molecular pattern production, our findings suggest that temperature oscillation might have driven dynamic co-evolution of distinct plant immune signaling responding to pathogen physiological changes. Innate immunity is triggered by the activation of immune receptors through the detection of non-self components. The first line of innate immunity is initiated by the detection of pathogen-associated molecular patterns or microbe-associated molecular patterns (MAMPs) through pattern-recognition receptors. In plants, MAMPs are perceived by cell-surface receptor-like kinases (RLKs) or receptor-like proteins to mount pattern-triggered immunity (PTI) [1] , [2] . Bacterial flagellin and elongation factor Tu are perceived by leucine-rich repeat RLK (LRR-RLK), FLS2 and EFR, respectively [3] , [4] . Upon ligand perception, FLS2 and EFR rapidly associate with another LRR-RLK BAK1, thereby initiating downstream signaling [5] , [6] . A receptor-like cytoplasmic kinase BIK1 is quickly phosphorylated upon flagellin or elongation factor Tu perception. BIK1 is associated with FLS2/BAK1 and EFR/BAK1 receptor complexes and is directly phosphorylated by BAK1 (refs 7 , 8 ). MAPK (mitogen-activated protein kinase) cascades and CDPKs (calcium-dependent protein kinases) act downstream of LRR-RLK receptor complexes in transducing intracellular signaling events, which ultimately lead to transcriptional reprogramming [9] , [10] . PTI signaling could be downregulated by the turnover of MAMP receptors. Two E3 ubiquitin ligases PUB12 and PUB13 interact with and ubiquitinate FLS2 receptor for proteosome-mediated degradation upon flagellin perception [11] . Adapted pathogens are able to suppress PTI by producing virulence effectors. In particular, many pathogenic bacteria deliver a plethora of effector proteins into host cells through type III secretion system (T3SS) to favour pathogen survival and multiplication and mediate effector-triggered susceptibility. Many of these effectors target important host components to sabotage host immune responses and physiology [12] , [13] , [14] . To confine or eliminate pathogens, plants further evolved intracellular nucleotide-binding domain leucine-rich repeat (NLR) proteins to directly or indirectly recognize effectors and initiate effector-triggered immunity (ETI) [15] , [16] . Plant NLR proteins share the structural similarity with mammalian NOD-like receptors that perceive intracellular MAMPs and danger signals to initiate inflammation and immunity [17] . Pseudomonas syringae effector AvrRpt2 is recognized by Arabidopsis NLR protein RPS2, whereas two sequence-unrelated effectors AvrRpm1 and AvrB are recognized by RPM1 to initiate ETI responses including transcriptional reprogramming and localized programmed cell death termed as hypersensitive response (HR). Instead of direct NLR–effector interaction, RPS2 and RPM1 monitor the perturbation of host protein RIN4 targeted by pathogen effectors to mount defense responses [18] , [19] . Specific calcium-dependent protein kinases downstream of NLR proteins sense sustained increase in cytosolic Ca 2+ concentration and regulate the bifurcate defense responses via phosphorylation of different substrates and subcellular dynamics [20] . Environmental factors often have profound impacts on microbial invasion and host evasion [21] . Temperature fluctuates both daily and seasonally and has long been considered as one of the key determinants for disease epidemics [22] , [23] . In many cases, virulence genes of mammalian pathogens are induced at 37 °C, which is a typical body temperature of mammalians, but are repressed below 30 °C (ref. 24 ). Accordingly, elevating mammalian body temperature to fever range results in an increase in MAMP-induced downstream signaling [25] . In contrast, many virulence determinants in plant pathogenic bacteria are induced at 16–24 °C and repressed at >28 °C (refs 26 , 27 , 28 ). For instance, P. syringae effectors HrmA and AvrPto were secreted at their highest amounts when the temperature was between 18 and 22 °C (ref. 26 ). The production of P. syringae phytotoxin coronatine is also temperature-sensitive: induced at 18 °C and repressed at 28 °C (ref. 29 ). Plant body temperature fluctuates with their living environment on a daily basis. It remains unknown whether and how plants integrate ambient temperature oscillation with regulation of inducible defense programs triggered by distinct pathogen components. Here we show that plant immunity is inextricably linked with ambient temperature changes. ETI signaling is preferentially activated at relatively low temperatures (10–23 °C), whereas PTI signaling is activated at moderately elevated temperatures (23–32 °C). The temperature preference for PTI and ETI signaling activation is coincident with the temperature effect on bacterial physiology: the elevated temperatures inhibit bacterial effector secretion but promote bacterial proliferation. The interplay between temperature and plant immunity is further supported by the enhanced PTI; however, reduced ETI responses in Arabidopsis arp6 and hta9hta11 mutants, which phenocopy plants grown at the elevated temperatures. Elevated temperatures promote PTI responses To monitor the specific immune responses at different ambient temperatures, we first tested the impact of different temperatures on PTI responses. Elicitation of PTI in Arabidopsis is accompanied by profound immune gene transcriptional reprogramming. The PTI marker genes WRKY29 and FRK1 were preferentially activated at the elevated ambient temperatures between 23 and 32 °C in response to flg22 (a 22-amino-acid peptide of bacterial flagellin) in Arabidopsis leaves or protoplasts ( Fig. 1a,b ). The optimal temperature for WRKY29 and FRK1 activation by flg22 was around 28 °C. The activation was dramatically reduced when the temperature was below 16 °C. Plants perceive a variety of MAMPs with different receptors. The similar temperature preference was observed for the activation of pWRKY29::LUC (the WRKY29 promoter fused with a luciferase reporter) by other MAMPs, including bacterial harpin Z (HrpZ), fungal chitin and oomycete necrosis-inducing Phytophthora protein 1 (NPP1) ( Fig. 1c ). Perception of different MAMPs elicits convergent early signaling events, including MAPK activation. The MAPK activation in seedlings treated with flg22 became gradually pronounced with the increased ambient temperatures ( Fig. 2a ). Apparently, the activation of MAPKs by flg22 at 28 or 23 °C occurred faster and stronger than that at 16 °C. Consistently, flg22-induced phosphorylation of BIK1 was largely reduced at 16 °C but increased at 28 °C ( Fig. 2b ). It is unlikely that the enhanced kinase activation results from the elevated protein synthesis at higher temperatures, as the samples were incubated at different temperatures for a relatively short time period (from 5 to 45 min with 15 min pretreatment). Thus, plants exhibit a preference to operate PTI responses at a relatively high ambient temperature above 23 °C. The in vitro bacterial growth assay indicates that bacterium P. syringae pv. tomato DC3000 ( Pst ) multiplies more vigorously at the elevated ambient temperatures above 23 °C than at temperatures below 16 °C ( Supplementary Fig. S1 ). The increased bacterial growth rate at the elevated ambient temperatures likely leads to the production of more MAMPs. 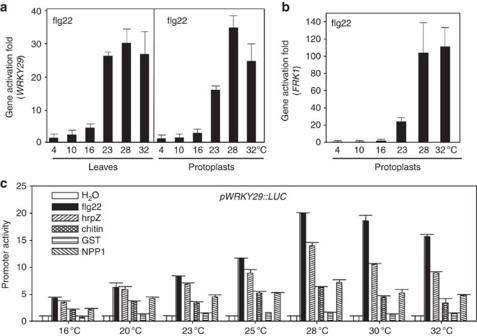Figure 1: Elevated temperatures promote gene activation in PTI signaling. (a) flg22-inducedWRKY29activation inArabidopsisleaves and protoplasts at different temperatures. Leaves or protoplasts from 4-week-old plants were treated with H2O or 100 nM flg22 for 3 h for RNA isolation and real-time RT-PCR (qRT-PCR) analysis. The expression ofWRKY29was normalized to the expression ofUBQ10. (b) flg22-inducedFRK1activation inArabidopsisprotoplasts at different temperatures. Protoplasts from 4-week-old plants were treated with H2O or 100 nM flg22 for 3 h for RNA isolation and qRT-PCR analysis. The expression ofFRK1was normalized to the expression ofUBQ10. The gene activation fold is presented as the ratio of flg22 treatment to H2O treatment with the mean±s.e.m. (n=3) from three independent biological replicates. (c) Activation ofpWRKY29::LUCby different MAMPs at different temperatures. The protoplasts were transfected withpWRKY29::LUCandpUBQ::GUSas an internal control and treated with 10 nM flg22, 10 nM HrpZ, 50 μg ml−1chitin, or 20 nM NPP1 for 3 h at the indicated temperatures. GST is the control for NPP1. The promoter activity was shown as the ratio of relative luciferase activity to GUS activity. The data are shown as mean±s.e.m. (n=3) from three independent biological replicates. The above experiments were repeated three times with similar results. Figure 1: Elevated temperatures promote gene activation in PTI signaling. ( a ) flg22-induced WRKY29 activation in Arabidopsis leaves and protoplasts at different temperatures. Leaves or protoplasts from 4-week-old plants were treated with H 2 O or 100 nM flg22 for 3 h for RNA isolation and real-time RT-PCR (qRT-PCR) analysis. The expression of WRKY29 was normalized to the expression of UBQ10 . ( b ) flg22-induced FRK1 activation in Arabidopsis protoplasts at different temperatures. Protoplasts from 4-week-old plants were treated with H 2 O or 100 nM flg22 for 3 h for RNA isolation and qRT-PCR analysis. The expression of FRK1 was normalized to the expression of UBQ10 . The gene activation fold is presented as the ratio of flg22 treatment to H 2 O treatment with the mean±s.e.m. ( n =3) from three independent biological replicates. ( c ) Activation of pWRKY29::LUC by different MAMPs at different temperatures. The protoplasts were transfected with pWRKY29::LUC and pUBQ::GUS as an internal control and treated with 10 nM flg22, 10 nM HrpZ, 50 μg ml −1 chitin, or 20 nM NPP1 for 3 h at the indicated temperatures. GST is the control for NPP1. The promoter activity was shown as the ratio of relative luciferase activity to GUS activity. The data are shown as mean±s.e.m. ( n =3) from three independent biological replicates. The above experiments were repeated three times with similar results. 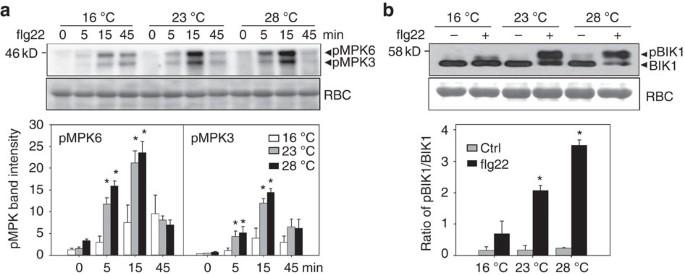Figure 2: Elevated temperatures promote early PTI signaling. (a) flg22-induced MAPK activation at different temperatures. Ten-day-old WT seedlings were treated with 100 nM flg22 at different temperatures for indicated time. MAPK activation was detected with an α-pERK antibody and Coomassie Brilliant Blue staining of Rubisco (RBC) protein is shown for equal loading control. (b) flg22-induced BIK1 phosphorylation in protoplasts at different temperatures. The band intensities of pMPK3, pMPK6, BIK1 and pBIK1 were quantified using the Image J software and presented with mean±s.e.m. (n=3) from three independent biological replicates. * indicates a significant difference withP<0.05 analysed with the SPSS software one-way ANOVA analysis when compared with corresponding data from 16 °C. The above experiments were repeated three times with similar results. Full size image Figure 2: Elevated temperatures promote early PTI signaling. ( a ) flg22-induced MAPK activation at different temperatures. Ten-day-old WT seedlings were treated with 100 nM flg22 at different temperatures for indicated time. MAPK activation was detected with an α-pERK antibody and Coomassie Brilliant Blue staining of Rubisco (RBC) protein is shown for equal loading control. ( b ) flg22-induced BIK1 phosphorylation in protoplasts at different temperatures. The band intensities of pMPK3, pMPK6, BIK1 and pBIK1 were quantified using the Image J software and presented with mean±s.e.m. ( n =3) from three independent biological replicates. * indicates a significant difference with P <0.05 analysed with the SPSS software one-way ANOVA analysis when compared with corresponding data from 16 °C. The above experiments were repeated three times with similar results. Full size image Elevated temperatures inhibit ETI responses Our finding is surprising, as it is generally believed that plant defense responses are inhibited at moderately elevated temperatures [30] . We further determined the temperature regulation of ETI responses triggered by P. syringae effector AvrRpt2. To avoid the complication of bacterial physiology, multiplication and effector secretion/delivery at different temperatures, we examined the immune responses in dexamethasone (Dex)-inducible AvrRpt2 transgenic plants [31] . Treatment with Dex induced the expression of the WRKY46 gene in Dex-AvrRpt2 plants [20] . Interestingly, the activation of WRKY46 by AvrRpt2 was also temperature sensitive ( Fig. 3a ). However, a distinct temperature preference was observed for ETI compared with PTI. The WRKY46 activation was detectable when temperature was as low as 4 °C, peaked at 16 °C, but was significantly attenuated when the temperature was >28 °C. A similar WRKY46 induction pattern was observed when AvrRpt2 was expressed in protoplasts at different temperatures ( Fig. 3a ). We also detected the temperature modulation of WRKY46 activation mediated by NLR protein RPM1 in response to P. syringae effector AvrRpm1 or AvrB ( Fig. 3b ). The optimal activation of WRKY46 by AvrRpm1 or AvrB was also observed at 16 °C, and the elevated temperatures suppressed WRKY46 activation. In addition, the AvrRpt2-mediated cell death in Dex-AvrRpt2 plants was significantly reduced at 28 °C and was almost completely abolished at 32 °C ( Fig. 3c ). Interestingly, cell death was clearly observed even at 4 °C. The avrRpt2 gene was expressed at a similar level after Dex treatment at different temperatures ( Fig. 3c ). The cell death induced by bacteria Pst carrying avrRpt2 was also inhibited at 32 °C ( Supplementary Fig. S2A ). Similarly, AvrRpm1- and AvrB-mediated cell death was significantly attenuated at the elevated temperatures when they were expressed in protoplasts ( Supplementary Fig. S2B ). The reduced activity of AvrRpt2, AvrRpm1 and AvrB at the elevated ambient temperatures was not because of the reduced protein expression ( Fig. 4a ). The data indicate that elevated temperatures could suppress Arabidopsis NLR protein RPM1 and RPS2-mediated ETI signaling. This observation is consistent with the finding that disease resistance and HR induced by Pst carrying avrRpt2 or avrRpm1 were reduced at 28 °C compared with that at 22 °C (ref. 30 ). 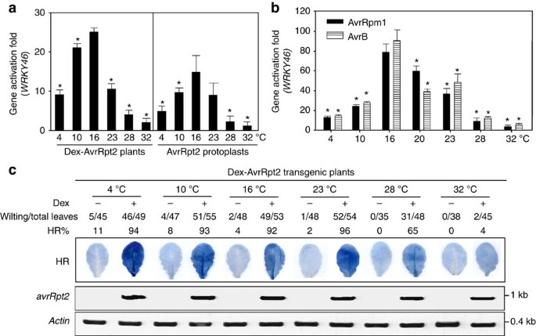Figure 3: Elevated temperatures inhibit ETI responses. (a) Activation ofWRKY46by AvrRpt2 at different temperatures. Four-week-oldDex-AvrRpt2plants were hand-inoculated with H2O or 10 μM Dex, or the protoplasts were transfected with AvrRpt2 or a vector control, and incubated at different temperatures for 6 h before sample collection for RNA isolation. The gene activation fold is presented as the ratio ofAvrRpt2expression to controls with the mean±s.e.m. (n=3) from three independent biological replicates. (b) Activation ofWRKY46by AvrRpm1 or AvrB at different temperatures. The protoplasts were transfected withAvrRpm1,AvrBor a vector control and incubated at different temperatures for 6 h before sample collection for RNA isolation. The data are shown as mean±s.e.m. (n=3) from three independent biological replicates. * indicates a significant difference withP<0.05 analysed with the SPSS software one-way ANOVA analysis when compared with corresponding data from 16 °C. (c) Cell death inDEX-avrRpt2transgenic plants at different temperatures. TheDEX-avrRpt2transgenic plants were hand-inoculated with H2O or 10 μM Dex and incubated at different temperatures. The cell death was recorded 24 hpi for plants incubated at 16, 23, 28 and 32 °C, 40 hpi for plants at 10 °C and 48 hpi for plants at 4 °C. The cell death was shown with Trypan blue staining and % indicates the percentage of wilting leaves of total inoculated leaves. The expression ofavrRpt2after DEX treatment is shown. Actin is the control for RT-PCR. The above experiments were repeated three times with similar results. Figure 3: Elevated temperatures inhibit ETI responses. ( a ) Activation of WRKY46 by AvrRpt2 at different temperatures. Four-week-old Dex-AvrRpt2 plants were hand-inoculated with H 2 O or 10 μM Dex, or the protoplasts were transfected with AvrRpt2 or a vector control, and incubated at different temperatures for 6 h before sample collection for RNA isolation. The gene activation fold is presented as the ratio of AvrRpt2 expression to controls with the mean±s.e.m. ( n =3) from three independent biological replicates. ( b ) Activation of WRKY46 by AvrRpm1 or AvrB at different temperatures. The protoplasts were transfected with AvrRpm1 , AvrB or a vector control and incubated at different temperatures for 6 h before sample collection for RNA isolation. The data are shown as mean±s.e.m. ( n =3) from three independent biological replicates. * indicates a significant difference with P <0.05 analysed with the SPSS software one-way ANOVA analysis when compared with corresponding data from 16 °C. ( c ) Cell death in DEX-avrRpt2 transgenic plants at different temperatures. The DEX-avrRpt2 transgenic plants were hand-inoculated with H 2 O or 10 μM Dex and incubated at different temperatures. The cell death was recorded 24 hpi for plants incubated at 16, 23, 28 and 32 °C, 40 hpi for plants at 10 °C and 48 hpi for plants at 4 °C. The cell death was shown with Trypan blue staining and % indicates the percentage of wilting leaves of total inoculated leaves. The expression of avrRpt2 after DEX treatment is shown. Actin is the control for RT-PCR. The above experiments were repeated three times with similar results. 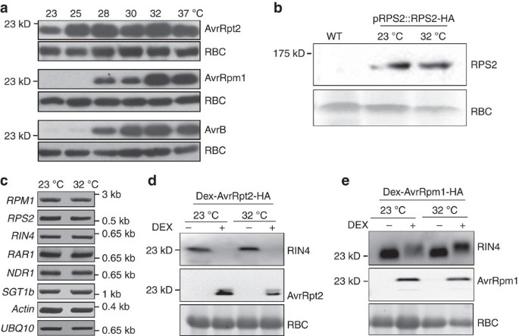Figure 4: Elevated temperatures do not suppress expression of bacterial effector and plant defense-related genes. (a) Expression of effector proteins at different temperatures. The protoplasts were transfected withAvrRpt2,AvrRpm1orAvrBand incubated at different temperatures for 6 h before sample collection for western blot with an α-HA antibody. Western blot with an α-RBC (Rubisco) antibody is shown as a loading control. (b) RPS2 protein level at 23 and 32 °C. ThepRPS2::RPS2-HAplants were incubated at 23 and 32 °C for 9 h before sample collection for western blot with an α-HA antibody. (c) Expression of plant resistance and signaling genes at 23 and 32 °C using RT-PCR analysis. The plants were incubated at 23 and 32 °C for 6 h before sample collection for RNA isolation. AvrRpt2-mediated RIN4 degradation (d) and AvrRpm1-mediated RIN4 phosphorylation (e) at different temperatures. Dex-AvrRpt2-HA (in Col-0 background) or Dex-AvrRpm1-HA transgenic plants (inrpm1background) were infiltrated with 10 μM Dex or H2O for 8 h. Immunoblot was performed with an α-RIN4 or α-HA antibody. Staining of RBC shows equal loading. The above experiments were repeated three times with similar results. Full size image Figure 4: Elevated temperatures do not suppress expression of bacterial effector and plant defense-related genes. ( a ) Expression of effector proteins at different temperatures. The protoplasts were transfected with AvrRpt2 , AvrRpm1 or AvrB and incubated at different temperatures for 6 h before sample collection for western blot with an α-HA antibody. Western blot with an α-RBC (Rubisco) antibody is shown as a loading control. ( b ) RPS2 protein level at 23 and 32 °C. The pRPS2::RPS2-HA plants were incubated at 23 and 32 °C for 9 h before sample collection for western blot with an α-HA antibody. ( c ) Expression of plant resistance and signaling genes at 23 and 32 °C using RT-PCR analysis. The plants were incubated at 23 and 32 °C for 6 h before sample collection for RNA isolation. AvrRpt2-mediated RIN4 degradation ( d ) and AvrRpm1-mediated RIN4 phosphorylation ( e ) at different temperatures. Dex-AvrRpt2-HA (in Col-0 background) or Dex-AvrRpm1-HA transgenic plants (in rpm1 background) were infiltrated with 10 μM Dex or H 2 O for 8 h. Immunoblot was performed with an α-RIN4 or α-HA antibody. Staining of RBC shows equal loading. The above experiments were repeated three times with similar results. Full size image Elevated temperature does not affect NLR and signaling gene expression The compromised NLR immune responses at the elevated temperatures could be a result of the reduced transcript/protein level of NLRs or other components in NLR signaling [32] . We compared the RPS2 protein level in pRPS2::RPS2-HA transgenic plants at 23 and 32 °C. The RPS2 protein level did not differ significantly in plants incubated at 32 °C for 9 h compared with that at 23 °C ( Fig. 4b ). Similarly, the transcripts of RPM1, RPS2, RIN4 , RAR1, NDR1 and SGT1b were comparable in plants incubated at 23 and 32 °C ( Fig. 4c , primer sequences are in Supplementary Table ). Thus, the short-term treatment with the elevated ambient temperatures unlikely changed NLR protein stability, signaling component transcripts or other plant physiology. However, we cannot rule out the possibility of other effects, such as differential subcellular localizations of NLR proteins caused by temperature changes. AvrRpt2 degrades Arabidopsis RIN4 protein to activate RPS2 signaling [18] , [19] . Apparently, the AvrRpt2-mediated RIN4 degradation still occurred at 28 and 32 °C, although the HR was significantly blocked at these elevated temperatures ( Fig. 4d and Supplementary Fig. S2C ). Similarly, AvrRpm1-mediated RIN4 phosphorylation as shown with a mobility shift seems not to be affected by the elevated temperature ( Fig. 4e ). The data suggest that the temperature operation of ETI responses occurs independent or downstream of RIN4 modification. Enhanced PTI responses in arp6 – 10 and hta9hta11 mutant plants Recent research has identified some important factors in response to ambient temperature changes in plants [33] . In particular, alternative histone H2A.Z nucleosomes are essential for Arabidopsis to precisely perceive ambient temperature and may function as an evolutionarily conserved thermosensor to regulate the ambient temperature transcriptome [34] . H2A.Z-containing nucleosomes wrap DNA more tightly than canonical H2A nucleosomes and can modulate transcription in a temperature-dependent manner. At elevated ambient temperature, H2A.Z nucleosome occupancy declines, which leads to the expression of warm-temperature-responsive genes. Consistently, in the absence of H2A.Z deposition, plants display constitutive warm-temperature responses [34] . The Arabidopsis mutants deficient in incorporating H2A.Z into the nucleosomes, such as arp6 and hta9hta11, phenocopy plants grown at the elevated ambient temperature and possess constitutive warm-temperature transcriptome [34] . We therefore determined the PTI and ETI responses in arp6 and hta9hta11 mutants. We first compared the flg22-induced MAPK activation in hta9hta11 and arp6 mutants at 23 °C. Apparently, the activation of MAPKs by flg22 was stronger in both hta9hta11 and arp6 mutants than that in wild-type (WT) plant seedlings, in particular 15 min after treatment ( Fig. 5a ). The induction of PTI marker genes, including FRK1 and At2g17740 , by flg22 treatment was also enhanced in hta9hta11 and/or arp6 mutants compared with that in WT seedlings ( Fig. 5b ). Consistent with the enhanced PTI responses, it has been reported that hta9hta11 mutant displayed enhanced resistance to Pst infection [35] . 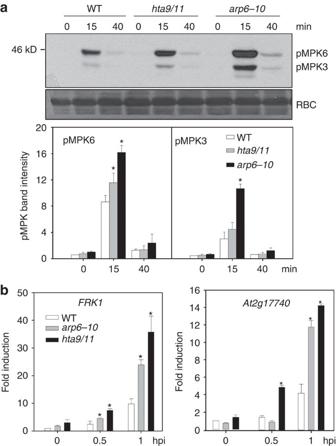Figure 5: Enhanced PTI responses inarp6–10andhta9hta11mutant plants. (a) flg22-induced MAPK activation in WT and mutants. Ten-day-old seedlings were treated with 100 nM flg22 at room temperature for indicated time. MAPK activation was detected with an α-pERK antibody. The band intensities of pMPK3 and pMPK6 were quantified using the Image J software and presented with mean±s.e.m. (n=3) from three independent biological replicates. * indicates a significant difference withP<0.05 analysed with the SPSS software one-way ANOVA analysis when compared with data from WT plants. (b) flg22-induced PTI marker gene expression. Ten-day-old seedlings of WT and mutants were treated with 100 nM flg22 for 0.5 or 1 h. The gene expression ofFRK1andAt2g17740was detected using qRT-PCR and normalized to the expression ofUBQ10. The data are shown as the mean±s.e.m. from three independent biological replicates. * indicates a significant difference withP<0.05 analysed with the SPSS software one-way ANOVA analysis when compared with data from WT plants. The above experiments were repeated three times with similar results. Figure 5: Enhanced PTI responses in arp6 – 10 and hta9hta11 mutant plants. ( a ) flg22-induced MAPK activation in WT and mutants. Ten-day-old seedlings were treated with 100 nM flg22 at room temperature for indicated time. MAPK activation was detected with an α-pERK antibody. The band intensities of pMPK3 and pMPK6 were quantified using the Image J software and presented with mean±s.e.m. ( n =3) from three independent biological replicates. * indicates a significant difference with P <0.05 analysed with the SPSS software one-way ANOVA analysis when compared with data from WT plants. ( b ) flg22-induced PTI marker gene expression. Ten-day-old seedlings of WT and mutants were treated with 100 nM flg22 for 0.5 or 1 h. The gene expression of FRK1 and At2g17740 was detected using qRT-PCR and normalized to the expression of UBQ10 . The data are shown as the mean±s.e.m. from three independent biological replicates. * indicates a significant difference with P <0.05 analysed with the SPSS software one-way ANOVA analysis when compared with data from WT plants. The above experiments were repeated three times with similar results. Full size image Reduced ETI responses in arp6 – 10 and hta9hta11 mutant plants In contrast to the enhanced PTI responses, the ETI responses were reduced in the hta9hta11 and arp6 mutants. The inoculation of Pst avrRpt2 or avrRpm1 at a relatively high inoculum elicits an HR in WT Arabidopsis plants. The leaves inoculated with Pst avrRpt2 show tissue collapse at about 12–24 h post inoculation ( hpi ), and the Pst avrRpm1- inoculated leaves show collapse at about 4–12 hpi . The progression of Pst avrRpt2- and avrRpm1 -triggered HR was slower in the hta9hta11 and arp6 mutants than that in WT plants ( Fig. 6a,b ). We also quantified HR using an electrolyte leakage assay. Consistently, compared with WT plants, hta9hta11 and arp6 mutants showed a compromised increase in conductance because of the release of electrolytes during cell death upon Pst avrRpt2 or avrRpm1 infection ( Fig. 6c,d ). The in planta bacterial multiplication of Pst avrRpt2 increased about 10-fold in the hta9hta11 and arp6 mutants compared with that in WT plants ( Fig. 7a ). The bacterial multiplication of Pst avrRpm1 increased about fivefold in the arp6 mutant compared with that in WT plants ( Fig. 7a ). The Pst avrRpt2 or avrRpm1 infection induces expression of several defense-related genes, such as AIG1 and PR1. The induction of AIG1 and PR1 by Pst avrRpt2 or avrRpm1 was significantly lower in hta9hta11 and arp6 mutants than that in WT plants ( Fig. 7b ). The data are consistent with the differential operation of two branches of plant innate immune signaling at different temperatures. 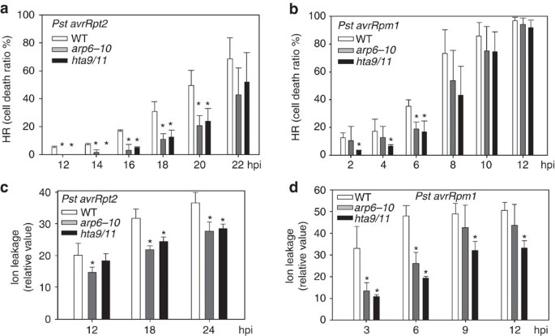Figure 6: Reduced ETI cell death inarp6–10andhta9hta11mutant plants. Compromised HR triggered byPst avrRpt2(a) andavrRpm1(b) inarp6–10andhta9/11mutant plants. Four-week-old WT and mutant plants were hand-inoculated with bacteria at a concentration of 1 × 108cfu ml−1. HR was examined by counting the percentage of wilting leaves of total inoculated leaves (>20) at different time points after inoculation. Electrolyte leakage induced byPst avrRpt2(c) andavrRpm1(d) was reduced inarp6–10andhta9/11mutant plants. Five leaf discs were excised from 4-week-old plants hand-inoculated with bacteria at 1 × 108cfu ml−1for each sample at each time point with three replicates. * indicates a significant difference withP<0.05 analysed with the SPSS software one-way ANOVA analysis when compared with data from WT plants. The data are shown as mean±s.e.m. (n=3) from three independent biological replicates. The data were analysed with the SPSS software one-way ANOVA analysis for statistical test. The above experiments were repeated three times with similar results. Figure 6: Reduced ETI cell death in arp6 – 10 and hta9hta11 mutant plants. Compromised HR triggered by Pst avrRpt2 ( a ) and avrRpm1 ( b ) in arp6 – 10 and hta9/11 mutant plants. Four-week-old WT and mutant plants were hand-inoculated with bacteria at a concentration of 1 × 10 8 cfu ml −1 . HR was examined by counting the percentage of wilting leaves of total inoculated leaves (>20) at different time points after inoculation. Electrolyte leakage induced by Pst avrRpt2 ( c ) and avrRpm1 ( d ) was reduced in arp6 – 10 and hta9/11 mutant plants. Five leaf discs were excised from 4-week-old plants hand-inoculated with bacteria at 1 × 10 8 cfu ml −1 for each sample at each time point with three replicates. * indicates a significant difference with P <0.05 analysed with the SPSS software one-way ANOVA analysis when compared with data from WT plants. The data are shown as mean±s.e.m. ( n =3) from three independent biological replicates. The data were analysed with the SPSS software one-way ANOVA analysis for statistical test. The above experiments were repeated three times with similar results. 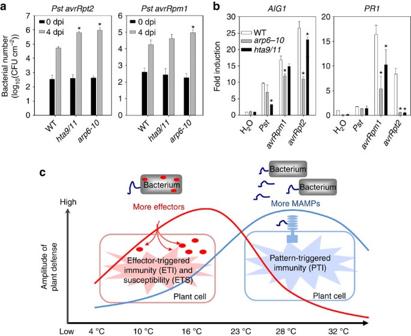Figure 7: Compromised ETI-mediated restriction of bacterial growth and defense gene activation inarp6–10andhta9hta11mutant plants. (a) Bacterial growth assay. Four-week-old plants were hand-inoculated withPst avrRpm1oravrRpt2at 5 × 105cfu ml−1. The bacterial growth was measured 0 days post inoculation (dpi) or 4 dpi. (b) ETI marker gene expression. Four-week-old plants were hand-inoculated with bacteria at 1 × 107cfu ml−1, and RNA was collected 6 hpi for qRT-PCR analysis. The expression ofAIG1andPR1was normalized to the expression ofUBQ10. The data are shown as the mean±s.e.m. (n=3) from three independent biological replicates and the asterisk (*) indicates a significant difference withP<0.05 analysed with the SPSS software one-way ANOVA analysis when compared with data from WT plants. (c) A model of temperature operation of distinct plant innate immune responses. At low ambient temperatures, bacteria secrete a large suite of virulence effectors to promote pathogenicity (ETS), which in turn stimulates plants to co-evolve and preferentially activate ETI signaling. At the elevated temperatures, bacteria multiply vigorously and produce increased amount of MAMPs, which stimulate plants to switch to PTI signaling. Ambient temperature fluctuation likely drives the dynamic co-evolution of bacterial pathogenesis and host immunity. The above experiments were repeated three times with similar results. Full size image Figure 7: Compromised ETI-mediated restriction of bacterial growth and defense gene activation in arp6 – 10 and hta9hta11 mutant plants. ( a ) Bacterial growth assay. Four-week-old plants were hand-inoculated with Pst avrRpm1 or avrRpt2 at 5 × 10 5 cfu ml −1 . The bacterial growth was measured 0 days post inoculation (dpi) or 4 dpi. ( b ) ETI marker gene expression. Four-week-old plants were hand-inoculated with bacteria at 1 × 10 7 cfu ml −1 , and RNA was collected 6 hpi for qRT-PCR analysis. The expression of AIG1 and PR1 was normalized to the expression of UBQ10 . The data are shown as the mean±s.e.m. ( n =3) from three independent biological replicates and the asterisk (*) indicates a significant difference with P <0.05 analysed with the SPSS software one-way ANOVA analysis when compared with data from WT plants. ( c ) A model of temperature operation of distinct plant innate immune responses. At low ambient temperatures, bacteria secrete a large suite of virulence effectors to promote pathogenicity (ETS), which in turn stimulates plants to co-evolve and preferentially activate ETI signaling. At the elevated temperatures, bacteria multiply vigorously and produce increased amount of MAMPs, which stimulate plants to switch to PTI signaling. Ambient temperature fluctuation likely drives the dynamic co-evolution of bacterial pathogenesis and host immunity. The above experiments were repeated three times with similar results. Full size image Microbe and host have co-evolved dynamically in their arms race for fitness and survival. Environmental factors often influence the physiological responses in both sides and have profound impacts on microbial pathogenesis and host immunity. In this study, we performed the quantitative assay of immune responses based on the activation of specific marker genes and found the differential temperature preference for the activation of two branches of plant innate immunity. Bacterial effector-triggered immune responses are preferentially activated at relatively low ambient temperatures, which are suitable for effector secretion, and are suppressed at the elevated ambient temperatures. The inhibition of ETI responses was not caused by the reduced expression of effectors, corresponding NLR receptors or known signaling components. In contrast, pattern-triggered immune responses are preferentially activated at the elevated ambient temperatures, which are optimal for bacterial growth, and are suppressed at low temperatures. Consistently, the immune responses of arp6 and hta9hta11 mutant plants, which are deficient in temperature sensing and phenocopy high-temperature-grown plants, mimic the responses of plants at the elevated temperatures with enhanced PTI signaling and yet reduced ETI signaling. Plant PTI signaling is initiated via cell-surface RLKs, whereas ETI signaling is mediated through intracellular NLR immune receptors. Although the precise mechanisms of how temperature sensing and signaling modulate the distinct plant immune responses are waiting to be elucidated, the differential temperature preferences of PTI and ETI responses suggest the distinct early signaling events downstream of cell-surface RLKs and intracellular NLR immune sensors. Our findings may have broad implication for agricultural practices to optimize plant immunity by considering the temperature-based defense strategies. Our study also provides insight into the effects of the current global climate change on plant disease management. Plant NLR proteins differ in the N -terminal domain and were further divided into coiled-coil (CC)-domain-containing- and Toll-interleukin-1 receptor (TIR)-domain-containing classes [17] , [36] . Growing evidence suggests the signaling activation in distinct subcellular compartments in TIR-NLR- and CC-NLR-mediated immunity [37] . In several cases, TIR-NLR-mediated immunity is temperature sensitive [38] , [39] , [40] , [41] . For instance, the tobacco mosaic virus resistance N gene- and Arabidopsis SNC1 gene-mediated responses are compromised at the elevated ambient temperatures above 28 °C (refs 38 , 39 ). Interestingly, suppressor screens and targeted mutagenesis suggest that SNC1 itself is a temperature-sensitive component of plant immune responses [42] . Several TIR-NLR immune receptors function in the nucleus [40] , [41] , [43] , [44] , whereas RPM1 and RPS2, the CC-NLR immune receptors, localize to the plasma membrane to initiate ETI signaling [18] , [45] . Our study indicates that RPM1- and RPS2-mediated responses are also largely compromised at temperatures >28 °C. Thus, both CC-NLR and TIR-NLR signaling pathways are modulated by ambient temperatures. Unexpectedly, we found that cell-surface-resident RLK-mediated PTI signalling is also temperature sensitive, with a pattern distinct from ETI signalling. In contrast to gradually compromised ETI responses, PTI responses become incrementally active with the elevated ambient temperatures ( Fig. 7c ). The differential temperature preference for the optimal operation of PTI and ETI signaling reconciles an enigmatic observation that the elevated temperatures inhibit bacterial effector secretion and yet promote bacterial proliferation [26] , [27] . Accordingly, plants have evolved combating mechanisms to maximize the PTI responses and turn down specific NLR-mediated responses to cope with a broad spectrum of microbial invasions at the elevated temperatures. At low ambient temperatures, bacteria secrete a large suite of virulence effectors to promote pathogenicity [26] , which in turn stimulates plants to co-evolve and preferentially activate ETI signaling ( Fig. 7c ). The primary function of these virulence effectors is to suppress PTI and induce effector-triggered susceptibility, which is accompanied with ETI in the plants carrying the corresponding receptors. Our results suggest that ambient temperature fluctuation drives the dynamic co-evolution of bacterial pathogenesis and host immunity, and plants integrate ambient temperature sensing to regulate two distinct branches of innate immunity mediated by cell-surface RLK and intracellular NLR immune sensors. ARP6 encodes a subunit of the evolutionarily conserved SWR1 complex that is necessary for inserting the alternative histone H2A.Z encoded by HTA gene family members into nucleosomes in place of H2A [34] , [35] . Arabidopsis arp6 and hta9hta11 mutants are deficient in incorporating histone H2A.Z into nucleosomes and display a constitutive warm-temperature transcriptome [34] . The finding that arp6 and hta9hta11 phenocopy the plants grown at high temperatures on immunity points at a possible link between temperature-driven immune responses and transcriptional changes. It will be interesting to test whether arp6 and hta9hta11 mutants could suppress the temperature-dependent cell death in snc1-1 , mekk1 and mpk4 mutants [39] , [46] . Notably, the hta9hta11 mutant also displayed constitutive expression of certain defense-related genes, spontaneous cell death and increased resistance to Pst infections, suggesting a link between H2A.Z-regulated gene expression and plant immunity [35] . Consistent with this observation, we showed that arp6 and hta9hta11 mutants have enhanced flg22-mediated responses. However, the ETI responses are suppressed in arp6 and hta9hta11 mutants, suggesting the opposite role of H2A.Z-containing nucleosomes in modulating PTI and ETI responses. Future study will uncover the molecular link between H2A.Z-mediated temperature perception and specific responses in ETI and PTI signaling. Plant growth conditions and temperature treatment Arabidopsis WT (Col-0), arp6 – 10 and hta9hta11 mutant plants were grown in pots containing soil (Metro Mix 360) in a growth room at 23 °C, 60% relative humidity and 75 μE m −2 s −1 light with a 12-h photoperiod for ~4 weeks before protoplast isolation, bacterial inoculation or different temperature treatments. The arp6 – 10 and hta9hta11 mutant seeds were obtained from Dr. P. Wigge of the John Innes Centre. To test temperature effects, plants were transferred to individual growth chambers set at different temperatures 15 min before treatments and treated for the indicated time. Bacterial inoculation assay Pst , Pst avrRpm1 or avrRpt2 strains were grown overnight at 28 °C in the KB medium containing rifamycin (50 μg ml −1 ) or in combination with kanamycin (50 μg ml −1 ). Bacteria were pelleted by centrifugation, washed and diluted to the desired density. The leaves were hand-inoculated with bacteria using a needleless syringe, collected at the indicated time for bacterial counting, cell death staining, electrolyte leakage assays or for RNA isolation. To measure bacterial growth, two leaf discs were ground in 100 μl H 2 O, and serial dilutions were plated on KB medium with appropriate antibiotics. Bacterial colony forming units (cfu) were counted 2 days after incubation at 28 °C. Each data point is shown as triplicates. At least three independent repeats were performed for all experiments. The representative data with similar results were shown. The statistical analysis was performed with the SPSS software one-way analysis of variance (ANOVA) analysis (SPSS Inc., Chicago). Protoplast transient assay Protoplast isolation and transient expression assays were conducted as described [7] , [20] . In general, 50 μl protoplasts at the density of 2 × 10 5 ml −1 and 10 μg DNA were used for promoter activity; 100 μl protoplasts and 20 μg DNA were used for protein expression; and 500 μl protoplasts and 100 μg DNA were used for RT-PCR analyses. For reporter assay, pUBQ10::GUS was cotransfected as an internal transfection control, and the promoter activity was presented as LUC/GUS ratio. Protoplasts transfected with empty vector were used as a control. MAPK activity and BIK1 phosphorylation assays To detect MAPK activity, 10-day-old WT, hta9/hta11 and arp6 – 10 seedlings grown on 1/2MS medium were transferred to water for overnight and then treated with 100 nM flg22 or H 2 O for indicated time points and frozen in liquid nitrogen. The seedlings were homogenized in an extraction buffer containing 50 mM Tris-HCl, pH7.5, 100 mM NaCl, 15 mM EGTA, 10 mM MgCl 2 , 1 mM NaF, 0.5 mM NaVO 3 , 30 mM β-glycerophosphate, 0.1% IGEPAL, 0.5 mM PMSF and 1% protease inhibitor cocktail. Equal amount of total protein was electrophoresed on 10% SDS–PAGE. An α-pERK antibody (1:2,000) (Cell Signaling) was used to detect phosphorylation status of MPK3 and MPK6 with an immunoblot. For different temperature treatments, the seedlings were pretreated at different temperatures for 15 min and then treated with 100 nM flg22 or H 2 O for 10 min. For BIK1 phosphorylation assay, Arabidopsis protoplasts were transfected with HA epitope-tagged BIK1 and incubated at room temperature for overnight, pretreated at 16, 23 or 28 °C for 15 min and then treated with 100 nM flg22 or H 2 O for 10 min. Total protein was separated using 10% SDS–PAGE gels followed by an α-HA immunoblot (1:2,000). Full blots are provided in Supplementary Figs S3–S7 . Cell death assays For HR assays, the leaves of 4-week-old plants were hand-inoculated with 10 μM DEX or different bacteria at 1 × 10 8 cfu ml −1 , and the cell death was calculated as the percentage of wilting leaves to total leaves inoculated. For trypan blue staining, leaves of DEX-AvrRpt2 plants were inoculated with H 2 O or 10 μM DEX and collected at 24 hpi after treatment. The leaves were stained with trypan blue in lactophenol (lactic acid:glycerol:liquid phenol:distilled water=1:1:1:1) solution, then destained with 95% ethanol/lactophenol solution and washed with 50% ethanol. For electrolyte leakage assays, five leaf discs (0.5 cm diameter) were excised from the WT or mutants infiltrated with bacteria and pre-floated in 10 ml of ddH 2 O for 10–15 min to eliminate wounding effect. The ddH 2 O was then changed and electrolyte leakage was measured using a conductivity meter (VWR; Traceable Conductivity Meter) at 12, 18 and 24 hpi for Pst avrRpt2 or 3, 6, 9 and 12 hpi for Pst avrRpm1 with three replicates per time point per sample. RT-PCR and qRT-PCR analyses Total RNA was isolated from leaves or protoplasts with TRIzol Reagent (Invitrogen). One microgram of total RNA was used for complementary DNA (cDNA) synthesis with oligo (dT) primer and reverse transcriptase (New England BioLabs). qRT-PCR analysis was carried out using iTaq SYBR green Supermix (Bio-Rad) supplemented with ROX in an ABI GeneAmp PCR System 9700. The expression of PTI and ETI marker genes was normalized to the expression of UBQ10 . The regular RT-PCR was performed with 35 cycles. The primer sequences are described in Supplementary Table S1 . How to cite this article: Cheng, C. et al . Plant immune response to pathogens differs with changing temperatures. Nat. Commun. 4:2530 doi: 10.1038/ncomms3530 (2013).